Microtubule acetylation amplifies p38 kinase signalling and anti-inflammatory IL-10 production Reversible acetylation of α-tubulin is an evolutionarily conserved modification in microtubule networks. Despite its prevalence, the physiological function and regulation of microtubule acetylation remain poorly understood. Here we report that macrophages challenged by bacterial lipopolysaccharides (LPS) undergo extensive microtubule acetylation. Suppression of LPS-induced microtubule acetylation by inactivating the tubulin acetyltransferase, MEC17, profoundly inhibits the induction of anti-inflammatory interleukin-10 (IL-10), a phenotype effectively reversed by an acetylation-mimicking α-tubulin mutant. Conversely, elevating microtubule acetylation by inhibiting the tubulin deacetylase, HDAC6, or stabilizing microtubules via Taxol stimulates IL-10 hyper-induction. Supporting the anti-inflammatory function of microtubule acetylation, HDAC6 inhibition significantly protects mice from LPS toxicity. In HDAC6-deficient macrophages challenged by LPS, p38 kinase signalling becomes selectively amplified, leading to SP1-dependent IL-10 transcription. Remarkably, the augmented p38 signalling is suppressed by MEC17 inactivation. Our findings identify reversible microtubule acetylation as a kinase signalling modulator and a key component in the inflammatory response. Acetylation on lysine (K) 40 of α-tubulin is an evolutionarily conserved modification controlled by the acetyltransferase MEC17 (also termed αTAT1) [1] , [2] and the deacetylase HDAC6 (refs 3 , 4 ). The prevalence and highly enriched distribution of α-tubulin acetylation in the microtubule network suggests a fundamental function of this modification [5] , [6] . Surprisingly, mice lacking MEC17 or HDAC6 are grossly normal despite a remarkable perturbation in microtubule acetylation [7] , [8] , [9] , [10] . α-tubulin acetylation on K40 is also dispensable in Tetrahymena [11] . Thus, under laboratory conditions, microtubule acetylation is neither essential for development nor survival. These unexpected findings raise the possibility that microtubule acetylation might be associated with stress or adaptive response that promotes post-embryonic fitness. The tubulin deacetylase, HDAC6, has emerged as a promising therapeutic target. Genetic and pharmacological inhibition of HDAC6 has been shown to suppress neurodegenerative disorders, enhance immune-modulatory activity and alleviate depressive behaviours in animal models [12] , [13] , [14] , [15] . Although enhanced tubulin acetylation is often cited as the basis for the observed beneficial effects, the evidence is largely indirect. The critical question of how microtubule acetylation might intersect with various disorders is also not understood. The growing list of HDAC6 substrates further suggests that additional mechanism independent of tubulin acetylation might be involved [16] . Identifying the relevant substrate and underlying mechanism in this context would be critical for devising HDAC6-targeted therapies. In this report, we present evidence that microtubule acetylation is a critical component of innate immunity. Microtubule acetylation is induced by bacterial lipopolysaccharides (LPS) treatment and selectively required for the production of the anti-inflammatory cytokine IL-10. Modulation of tubulin acetylation by targeting MEC17 and HDAC6 profoundly affects IL-10 production and anti-inflammatory activity in macrophages and in mice. We further show that microtubule acetylation selectively enhances p38 signalling, leading to SP-1 dependent IL-10 transcription. Our study identifies acetylated microtubules as a signal amplifier and a key target in HDAC6-targeted therapies. HDAC6 deficiency leads to hyper-induction of IL-10 Innate immunity is critical for host defence against infectious agents but dispensable in a controlled laboratory environment. We therefore considered a potential role for microtubule acetylation in innate immune response. Macrophages are the key components in innate immunity by producing inflammatory cytokines and presenting foreign antigens. To investigate whether microtubule acetylation regulates macrophage function, we constructed macrophage lines (Raw264.7) with stable knockdown of HDAC6 by shRNAs ( Fig. 1a ) and assessed their ability to produce inflammatory cytokines upon bacterial LPS challenge. We found that HDAC6 knockdown (KD) modestly reduced the production of pro-inflammatory cytokines, TNF-alpha and IL-1beta ( Fig. 1b ) as well as IL-6 ( Supplementary Fig. 1a ). In stark contrast, the production of anti-inflammatory IL-10 was dramatically elevated in HDAC6 KD macrophages, more than fivefold higher than control macrophages ( Fig. 1c ). To confirm this finding, we examined bone marrow-derived macrophages isolated from HDAC6 knockout (KO) mice. A similar hyper-induction of IL-10 ( Fig. 1d ), but minor changes in pro-inflammatory cytokines ( Supplementary Fig. 1b ), was observed in HDAC6 KO primary macrophages treated with LPS. Importantly, LPS treatment also induced higher levels of serum IL-10 in HDAC6 KO mice than wild type mice in vivo ( Fig. 1e ). These results show that HDAC6 regulates IL-10 production induced by LPS. 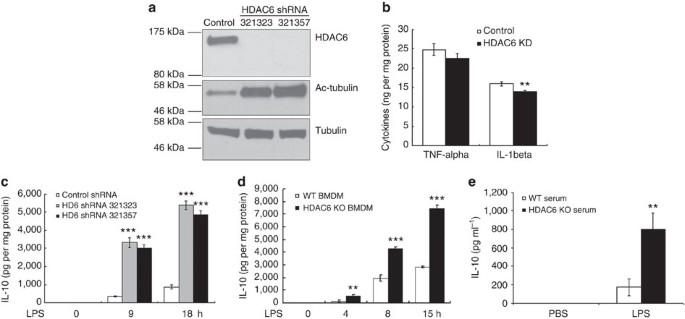Figure 1: LPS induced hyper-induction of IL-10 in HDAC6-deficient macrophages and mice. (a) HDAC6 was stably knocked down in macrophages (RAW264.7 cells) by two different HDAC6 shRNAs (no. 321323 and no. 321357). The levels of HDAC6 protein and α-tubulin acetylation were determined by immunoblotting. (b,c) Control and HDAC6 KD (shRNA 321323) macrophages were treated with LPS (1 μg ml−1) for 18 h and medium was subjected to ELISA for TNF-alpha and IL-1beta (b) and IL-10 production (c).HDAC6 KD by either shRNA significantly enhanced IL-10 production. The graph shows the means with s.e.m. (error bars) from three experiments. Asterisks indicate statistical significance (**P<0.01 and ***P<0.001, Student’st-test). (d) Bone marrow-derived primary macrophages (BMDM) isolated from WT and HDAC6 KO mice were treated with LPS (1 μg ml−1) for indicated time and medium was assayed for IL-10 levels by ELISA. HDAC6 KO BMDM produced significantly more IL-10 production compared to WT macrophages. The graph shows the means with s.e.m. (error bars) from three experiments. Asterisks indicate statistical significance (**P<0.01 and ***P<0.001, Student’st-test). (e) WT and HDAC6 KO mice were challenged by LPS (50 μg per mouse) through intraperitoneal (i.p.) injection and serum was analysed for IL-10 at 4 h post injection. Without LPS injection (PBS injection), IL-10 was not detectible. The graph shows the means with s.e.m. (error bars). Asterisks indicate statistical significance (**P<0.01, Student’st-test). Figure 1: LPS induced hyper-induction of IL-10 in HDAC6-deficient macrophages and mice. ( a ) HDAC6 was stably knocked down in macrophages (RAW264.7 cells) by two different HDAC6 shRNAs (no. 321323 and no. 321357). The levels of HDAC6 protein and α-tubulin acetylation were determined by immunoblotting. ( b , c ) Control and HDAC6 KD (shRNA 321323) macrophages were treated with LPS (1 μg ml −1 ) for 18 h and medium was subjected to ELISA for TNF-alpha and IL-1beta ( b ) and IL-10 production ( c ).HDAC6 KD by either shRNA significantly enhanced IL-10 production. The graph shows the means with s.e.m. (error bars) from three experiments. Asterisks indicate statistical significance (** P <0.01 and *** P <0.001, Student’s t -test). ( d ) Bone marrow-derived primary macrophages (BMDM) isolated from WT and HDAC6 KO mice were treated with LPS (1 μg ml −1 ) for indicated time and medium was assayed for IL-10 levels by ELISA. HDAC6 KO BMDM produced significantly more IL-10 production compared to WT macrophages. The graph shows the means with s.e.m. (error bars) from three experiments. Asterisks indicate statistical significance (** P <0.01 and *** P <0.001, Student’s t -test). ( e ) WT and HDAC6 KO mice were challenged by LPS (50 μg per mouse) through intraperitoneal (i.p.) injection and serum was analysed for IL-10 at 4 h post injection. Without LPS injection (PBS injection), IL-10 was not detectible. The graph shows the means with s.e.m. (error bars). Asterisks indicate statistical significance (** P <0.01, Student’s t -test). Full size image LPS-induced IL-10 requires MEC17 and α-tubulin acetylation We found that the hyper-induction of IL-10 in HDAC6 KD macrophages can be effectively suppressed by the re-introduction of a wild type but not c atalytic i nactive (Ci) mutant HDAC6, indicating that the deacetylase activity of HDAC6 is required for regulating IL-10 production ( Supplementary Fig. 1c,d ). Supporting this notion, treatment with an HDAC6-selective inhibitor, Tubastatin A (TBSA [17] ), strongly elevated IL-10 production in Raw264.7 induced by LPS ( Fig. 2a ). We next investigated whether microtubule acetylation is involved in IL-10 production. We assessed microtubule acetylation by staining LPS-activated macrophages with an acetylated α-tubulin-specific antibody [18] . This staining revealed a time-dependent increase in acetylated microtubules following LPS treatment ( Fig. 2b ). Immuno-blotting confirmed that microtubule acetylation was indeed induced by LPS treatment (Ac-tubulin, Fig. 2c ). Interestingly, LPS also caused a parallel increase in the tubulin acetyltransferase MEC17, whereas the deacetylase HDAC6 was largely unaffected ( Fig. 2c ). Thus, LPS induces MEC17 and microtubule acetylation in activated macrophages. 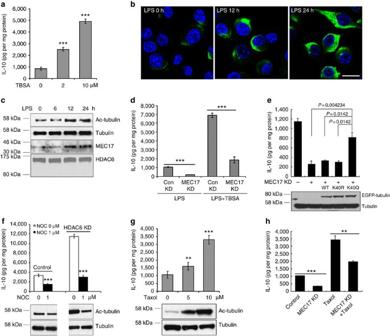Figure 2: α-tubulin acetylation activates LPS-induced IL-10 production in macrophages. (a) Macrophages (RAW264.7) were pretreated with a HDAC6 inhibitor, Tubastatin A (TBSA), at indicated doses for 12 h and followed by LPS (1 μg ml−1) treatment for 18 h. Medium was subjected to ELISA for IL-10 production. TBSA treatment markedly increased LPS-induced IL-10 production in a dose-dependent manner. (b) Macrophages were stained with an acetylated α-tubulin-specific antibody after LPS treatment at the indicated time. Immuno-staining showed that LPS treatment increased acetylated microtubules (green: Ac-tubulin; blue: DAPI; scale bar, 10 μM). (c) Macrophages were treated with LPS and analysed for acetylated tubulin, MEC17 and HDAC6 protein levels at indicated time. (d) MEC17 KD and control macrophages were pretreated with or without TBSA (10 μM) for 4 h and followed by LPS treatment for 18 h. Medium was harvested for IL-10 assay. Note that MEC17 KD strongly inhibited IL-10 production. (e) MEC17 KD macrophages were electroporated with pcDNA -EGFP, -EGFP-α-tubulin WT, K40→R and K40→Q mutant plasmids. Twenty four hours after transfection, cells were treated with LPS (1 μg ml−1) for 18 h and medium was subjected to IL-10 analysis. The graph shows the means with s.e.m. (error bars) from three experiments (Student’st-test). (f) HDAC6 KD and control macrophages were pretreated with nocodazole (NOC) for 4 h followed by another 18-h LPS treatment. NOC treatment reduced α-tubulin acetylation (bottom panel: immuno-blotting) and significantly blunted LPS-induced IL-10 levels in control and HDAC6 KD macrophages (upper panel: ELISA). (g) Macrophages were pretreated with microtubule-stabilizing agent, Taxol, for 4 h and then followed by another 18-hours LPS treatment. Taxol treatment led to a dose-dependent increase in α-tubulin acetylation (bottom panel: immuno-blotting) and a higher induction of IL-10 (upper panel: ELISA). (h) MEC17 KD macrophages were pretreated with Taxol for 4 h and followed by 18 h of LPS treatment. MEC17 KD significantly reduced Taxol-induced IL-10 production. For all ELISA assay, the graph shows the means with s.e.m. (error bars) from three experiments. Asterisks indicate statistical significance (**P<0.01 and ***P<0.001, Student’st-test). Figure 2: α-tubulin acetylation activates LPS-induced IL-10 production in macrophages. ( a ) Macrophages (RAW264.7) were pretreated with a HDAC6 inhibitor, Tubastatin A (TBSA), at indicated doses for 12 h and followed by LPS (1 μg ml −1 ) treatment for 18 h. Medium was subjected to ELISA for IL-10 production. TBSA treatment markedly increased LPS-induced IL-10 production in a dose-dependent manner. ( b ) Macrophages were stained with an acetylated α-tubulin-specific antibody after LPS treatment at the indicated time. Immuno-staining showed that LPS treatment increased acetylated microtubules (green: Ac-tubulin; blue: DAPI; scale bar, 10 μM). ( c ) Macrophages were treated with LPS and analysed for acetylated tubulin, MEC17 and HDAC6 protein levels at indicated time. ( d ) MEC17 KD and control macrophages were pretreated with or without TBSA (10 μM) for 4 h and followed by LPS treatment for 18 h. Medium was harvested for IL-10 assay. Note that MEC17 KD strongly inhibited IL-10 production. ( e ) MEC17 KD macrophages were electroporated with pcDNA -EGFP, -EGFP-α-tubulin WT, K40→R and K40→Q mutant plasmids. Twenty four hours after transfection, cells were treated with LPS (1 μg ml −1 ) for 18 h and medium was subjected to IL-10 analysis. The graph shows the means with s.e.m. (error bars) from three experiments (Student’s t -test). ( f ) HDAC6 KD and control macrophages were pretreated with nocodazole (NOC) for 4 h followed by another 18-h LPS treatment. NOC treatment reduced α-tubulin acetylation (bottom panel: immuno-blotting) and significantly blunted LPS-induced IL-10 levels in control and HDAC6 KD macrophages (upper panel: ELISA). ( g ) Macrophages were pretreated with microtubule-stabilizing agent, Taxol, for 4 h and then followed by another 18-hours LPS treatment. Taxol treatment led to a dose-dependent increase in α-tubulin acetylation (bottom panel: immuno-blotting) and a higher induction of IL-10 (upper panel: ELISA). ( h ) MEC17 KD macrophages were pretreated with Taxol for 4 h and followed by 18 h of LPS treatment. MEC17 KD significantly reduced Taxol-induced IL-10 production. For all ELISA assay, the graph shows the means with s.e.m. (error bars) from three experiments. Asterisks indicate statistical significance (** P <0.01 and *** P <0.001, Student’s t -test). Full size image To investigate whether MEC17 plays a role in IL-10 production, we knocked down MEC17 by two different shRNAs. Both MEC17 shRNAs led to a reduction in α-tubulin acetylation as expected ( Supplementary Fig. 2a ). Importantly, this was accompanied by a strong decrease in IL-10 production in TBSA-treated ( Fig. 2d ) or HDAC6 KD macrophages challenged by LPS ( Supplementary Fig. 2c ). Similar to HDAC6 inactivation, MEC17 KD had only a modest effect on pro-inflammatory cytokine production ( Supplementary Fig. 2d–f ). Interestingly, MEC17 KD also inhibited IL-10 production in control macrophages, indicating that MEC17 is a normal regulatory component in IL-10 production induced by LPS ( Fig. 2d , first two columns, Supplementary Fig. 2b ). Collectively, these results demonstrate an opposing activity of MEC17 and HDAC6 in IL-10 induction by LPS, thereby implicating microtubule acetylation in the regulation of anti-inflammatory IL-10 production. In addition to α-tubulin, HDAC6 has other substrates [19] , [20] , [21] . To substantiate that HDAC6 and MEC17 regulate IL-10 production via microtubule acetylation, we took two additional approaches. First, if MEC17 controls IL-10 production by catalysing α-tubulin acetylation, over-expression of an acetylation-mimicking α-tubulin should complement MEC17 knockdown and restore IL-10 production. Molecular modelling indicates that K40→Q (glutamine) mutation could mimic acetylation by promoting the formation of microtubule interprotofilament salt bridges [22] . We electroporated expression plasmids encoding for wild-type, acetylation-mimicking K40→Q, or acetylation-deficient K40→R α-tubulin into MEC17 KD cells followed by LPS treatment. Both K40→Q and K40→R α-tubulin mutants can be effectively incorporated into the microtubule network [23] . As shown in Fig. 2e ), over-expression of the acetylation-mimicking K40→Q, but not acetylation-deficient K40→R, α-tubulin mutant significantly restored IL-10 production in MEC17 KD cells. These results indicate that MEC17 regulates IL-10 production by increasing microtubule acetylation. Second, we took advantage of the observation that stable microtubules are more heavily acetylated [5] . Accordingly, we treated macrophages with a microtubule-destabilizing agent, nocodazole, and a stabilizing drug, Taxol, to decrease and increase microtubule acetylation, respectively. We found that nocodazole treatment reduced α-tubulin acetylation ( Fig. 2f ) and significantly blunted LPS-induced IL-10 production in both wild-type and HDAC6 KD macrophages ( Fig. 2f ). In contrast, Taxol treatment led to a dose-dependent increase in α-tubulin acetylation, which was accompanied by a higher induction of IL-10 ( Fig. 2g ). Importantly, the effect of Taxol on IL-10 production can be significantly reversed by MEC17 knockdown ( Fig. 2h ). Neither nocodazole nor Taxol treatment markedly affected the production of pro-inflammatory TNF-alpha, IL-6 or IL-1beta ( Supplementary Fig. 3 ). These results show that LPS-induced IL-10 production is positively regulated by the build-up of acetylated microtubules. α-tubulin acetylation amplifies LPS-induced p38 MAPK signal IL-10 production is regulated by the MAP kinases p38 and ERK, which activate IL-10 gene transcription (reviewed in ref. 24 ). We next sought to determine whether microtubule acetylation affects MAPK signalling linked to IL-10 production. LPS treatment induced transient phosphorylation and activation of p38, ERK and JNK ( Fig. 3a,b , lanes 1–6), as was previously reported [25] . Remarkably, we found that inhibition of HDAC6 by TBSA markedly increased the intensity and duration of LPS-induced p38 phosphorylation ( Fig. 3a , compare lanes 1–6 and 7–12). In contrast, TBSA only modestly affected phosphorylation of ERK1/2 and JNK ( Fig. 3b ). Robust and prolonged p38 phosphorylation was also observed in HDAC6 KO primary macrophages challenged by LPS ( Supplementary Fig. 4a ). Most importantly, the augmented p38 phosphorylation caused by TBSA was abrogated by MEC17 knockdown ( Fig. 3a , lanes 19–24). MEC17 knockdown, in fact, also reduced phosphorylated p38, but not ERK or JNK, in control macrophages challenged by LPS ( Fig. 3a , lanes 13–18), further supporting a specific regulatory role of microtubule acetylation in LPS-induced p38 signalling. Consistent with these findings, production of IL-10 in HDAC6 KD macrophages was strongly suppressed by a p38 inhibitor (SB202190) but not a JNK inhibitor (SP600125, Fig. 3c,d ). These results indicate that microtubule acetylation positively and specifically amplifies p38 kinase signalling and stimulates IL-10 production. 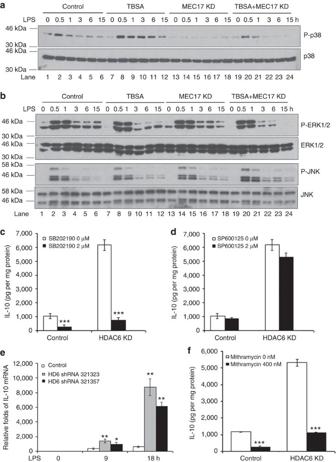Figure 3: Acetylation of α-tubulin regulates LPS-induced p38 signalling. (a,b) Control and MEC17 KD macrophages (RAW264.7) were treated with TBSA or DMSO for 12 h followed by LPS treatment for indicated time. p38 phosphorylation (a) and ERK1/2 and JNK phosphorylation (b) were determined by immuno-blotting. (c) Control and HDAC6 KD macrophages were pretreated with a p38 specific inhibitor, SB202190 (2 μM) or DMSO for 4 h and followed by 18 h of LPS treatment. p38 inhibitor treatment inhibited LPS-induced IL-10 production in control and HDAC6 KD macrophages in a dose-dependent manner. The graph shows the means with s.e.m. (error bars) from three experiments. Asterisks indicate statistical significance (***P<0.001, Student’st-test). (d) A JNK specific inhibitor, SP600125, had very limited effect on LPS-induced IL-10 production. The graph shows the means with s.e.m. (error bars) from three experiments. (e) Control and HDAC6 KD macrophages were treated with LPS for the indicated time and samples were subjected to IL-10 mRNA expression analysis by real-time PCR. HDAC6 KD significantly enhanced IL-10 mRNA upon LPS stimulation. The graph shows the means with s.e.m. (error bars) from three experiments. Asterisks indicate statistical significance (*P<0.05 and **P<0.005, Student’st-test). (f) HDAC6 KD and control macrophages were pretreated with the Sp1-specific inhibitor, mithramycin, for 6 h followed by 18 h of LPS treatment. ELISA analysis showed mithramycin treatment dramatically inhibited LPS-induced IL-10 production in control macrophages and HDAC6 KD macrophages. The graph shows the means with s.e.m. (error bars) from three experiments. Asterisks indicate statistical significance (***P<0.001, Student’st-test). Figure 3: Acetylation of α-tubulin regulates LPS-induced p38 signalling. ( a , b ) Control and MEC17 KD macrophages (RAW264.7) were treated with TBSA or DMSO for 12 h followed by LPS treatment for indicated time. p38 phosphorylation ( a ) and ERK1/2 and JNK phosphorylation ( b ) were determined by immuno-blotting. ( c ) Control and HDAC6 KD macrophages were pretreated with a p38 specific inhibitor, SB202190 (2 μM) or DMSO for 4 h and followed by 18 h of LPS treatment. p38 inhibitor treatment inhibited LPS-induced IL-10 production in control and HDAC6 KD macrophages in a dose-dependent manner. The graph shows the means with s.e.m. (error bars) from three experiments. Asterisks indicate statistical significance (*** P <0.001, Student’s t -test). ( d ) A JNK specific inhibitor, SP600125, had very limited effect on LPS-induced IL-10 production. The graph shows the means with s.e.m. (error bars) from three experiments. ( e ) Control and HDAC6 KD macrophages were treated with LPS for the indicated time and samples were subjected to IL-10 mRNA expression analysis by real-time PCR. HDAC6 KD significantly enhanced IL-10 mRNA upon LPS stimulation. The graph shows the means with s.e.m. (error bars) from three experiments. Asterisks indicate statistical significance (* P <0.05 and ** P <0.005, Student’s t -test). ( f ) HDAC6 KD and control macrophages were pretreated with the Sp1-specific inhibitor, mithramycin, for 6 h followed by 18 h of LPS treatment. ELISA analysis showed mithramycin treatment dramatically inhibited LPS-induced IL-10 production in control macrophages and HDAC6 KD macrophages. The graph shows the means with s.e.m. (error bars) from three experiments. Asterisks indicate statistical significance (*** P <0.001, Student’s t -test). Full size image Real-time PCR analysis showed that hyper-induction of IL-10 in HDAC6 deficient cells at the mRNA level ( Fig. 3e ). p38 promotes IL-10 production, at least in part, via the transcription factor Sp1 (ref. 26 ). We found that an Sp1 inhibitor, mithramycin, strongly suppressed IL-10 production in both control and HDAC6 deficient macrophages ( Fig. 3f ). Mithramycin only modestly affected TNF-alpha, IL-1beta and IL-6 production ( Supplementary Fig. 4b–d ), providing further evidence that the acetylated microtubule-p38-Sp1 signalling axis selectively regulates IL-10 production. In contrast to Sp1, inactivation of the AP1 transcription factor had a much weaker effect on IL-10 production ( Supplementary Fig. 5 ), consistent with a previous report [26] . These results provide evidence that MEC17/HDAC6-dependent microtubule acetylation modulates the strength of p38 signalling, which in turn, determines SP1-dependent transcriptional induction of IL-10. HDAC6 inhibition protects mice from acute toxicity of LPS The induction of IL-10 is critical for down-modulating pro-inflammatory response and preventing tissue injury caused by excessive inflammation (reviewed in ref. 24 ). Accordingly, an enhancement of IL-10 production by HDAC6 inactivation should dampen LPS-induced inflammation and toxicity in mice. To test this possibility, we injected C57BL6 mice with a dose of LPS that would typically cause cytokine storm and lethality alone or in conjunction with TBSA. As shown in Fig. 4a , mice that received TBSA showed much higher serum IL-10 levels after LPS treatment. Interestingly, TNF-alpha, IL-6 and IL-1beta levels were all reduced ( Fig. 4b–d ), supporting the anti-inflammatory activity of TBSA in vivo . Importantly, mice that received TBSA had a significantly higher survival rate compared with WT mice at all time points examined ( Fig. 4e ). Similar cytokine profile and survival advantage were also observed in HDAC6 KO mice treated with LPS ( Supplementary Fig. 6 ). These results demonstrate that HDAC6 inhibition can enhance anti-inflammatory activity and reduce LPS toxicity in vivo . 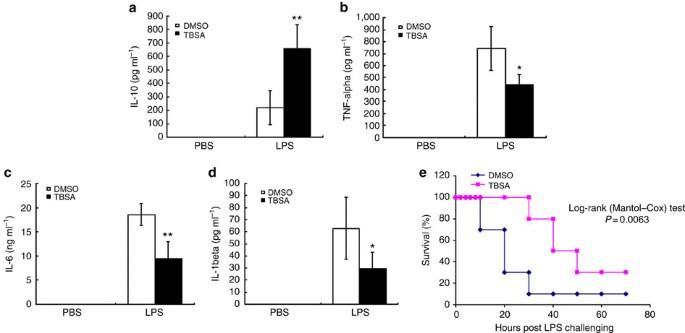Figure 4: Pharmacological inhibition of HDAC6 protects mice from LPS-induced acute inflammation. (a–d) TBSA treatment modified LPS-triggered production of IL-10, TNF-alpha, IL-6 and IL-1betain vivo. Male C57BL/6 mice were injected with either TBSA (0.5 mg per kg) or vehicle DMSO by daily i.p. for 7 days, followed by i.p. injection of LPS (50 μg per mouse) or vehicle PBS (five mice per group). After 4 h, serum samples were harvested and cytokine concentrations were measured by ELISA. LPS-induced IL-10 levels in serum were markedly increased in TBSA-injected mice, compared with DMSO vehicle injection (a). LPS-triggered TNF-alpha (b), IL-6 (c) and IL-1beta (d) levels in serum were decreased in TBSA-injected mice, compared with DMSO-injected mice. The graph shows the means with s.e.m. (error bars). Asterisks indicate statistical significance (*P<0.05 and **P<0.01, Student’st-test). (e) Mice were injected with TBSA (0.5 mg per kg) or vehicle DMSO by daily i.p. for 7 days followed by PBS or LPS (5 mg per kg) i.p. injection once. For the first 10 h post LPS challenge, survival was checked every 2 h. Afterwards, the survival was checked every 10 h. Survival curves showed a significant difference between DMSO and TBSA-treated mice (log-rank analysisP<0.01;n=10 in each group). Figure 4: Pharmacological inhibition of HDAC6 protects mice from LPS-induced acute inflammation. ( a – d ) TBSA treatment modified LPS-triggered production of IL-10, TNF-alpha, IL-6 and IL-1beta in vivo . Male C57BL/6 mice were injected with either TBSA (0.5 mg per kg) or vehicle DMSO by daily i.p. for 7 days, followed by i.p. injection of LPS (50 μg per mouse) or vehicle PBS (five mice per group). After 4 h, serum samples were harvested and cytokine concentrations were measured by ELISA. LPS-induced IL-10 levels in serum were markedly increased in TBSA-injected mice, compared with DMSO vehicle injection ( a ). LPS-triggered TNF-alpha ( b ), IL-6 ( c ) and IL-1beta ( d ) levels in serum were decreased in TBSA-injected mice, compared with DMSO-injected mice. The graph shows the means with s.e.m. (error bars). Asterisks indicate statistical significance (* P <0.05 and ** P <0.01, Student’s t -test). ( e ) Mice were injected with TBSA (0.5 mg per kg) or vehicle DMSO by daily i.p. for 7 days followed by PBS or LPS (5 mg per kg) i.p. injection once. For the first 10 h post LPS challenge, survival was checked every 2 h. Afterwards, the survival was checked every 10 h. Survival curves showed a significant difference between DMSO and TBSA-treated mice (log-rank analysis P <0.01; n =10 in each group). Full size image Despite its prevalence and conservation, the physiological function of acetylated microtubules has been elusive. Our study has provided evidence that microtubule acetylation is a critical regulatory component for p38 kinase signalling in macrophages. The build-up of acetylated microtubules in response to LPS augments and sustains p38 signalling that stimulates anti-inflammatory IL-10 production. Since microtubule acetylation does not directly affect the production of key pro-inflammatory cytokines ( Fig. 1b , Supplementary Figs 2 and 3 ), these findings suggest that HDAC6 inhibitors would promote natural resolution of pathological inflammation by stimulating IL-10 production while permitting the initiation of pro-inflammatory response. Indeed, we found that TBSA treatment significantly protects mice from inflammatory shock induced by LPS ( Fig. 4 ). The increase in IL-10 production could potentially contribute to the reported neuro-protective and anti-depressive effects of HDAC6 inhibition where inflammation is known to be a pathogenic factor [27] , [28] . Of interest, HDAC6-deficient T regulatory cells are more active than their wild-type counterparts in suppressing T effector cell proliferation [16] . Whether microtubule acetylation also plays a similar regulatory role in adaptive immunity is a critical issue to be determined. Our study identifies p38 signalling as a key downstream effector of microtubule acetylation in macrophages ( Fig. 3a ), whereas JNK signalling is largely independent of microtubule acetylation ( Fig. 3b ). In macrophages, acetylated microtubules might be considered a unique ‘signal amplifier’ where selective signalling events can be maintained and propagated. This proposition raises a possibility that axons and primary cilia, which are highly enriched for acetylated microtubules [29] , [30] , might use a similar mechanism to propagate selective signalling events. How microtubule acetylation selectively affects p38 signalling remains to be determined. Intriguingly, lysine 40 of α-tubulin is located inside the microtubule lumen and its acetylation increases the size of the lumen [22] , [31] , [32] . The finding that K40 acetylation-mimicking α-tubulin mutant can restore IL-10 production in MEC17-deficient cells ( Fig. 2e ) suggests that luminal dimension of microtubules could potentially affect p38 signalling. Whether the p38-signalling complex can enter the lumen of acetylated microtubules and signal from within is of great interest in the future. Antibodies and reagents The following antibodies were used for western blot: p-ERK1/2 (#4370, 1:2,000), ERK1/2 (#9102, 1:1,000), p-JNK (#4668, 1:1,000), JNK (#9258, 1:1,000), p-p38 (#4511, 1;1,000), and p38 (#9212, 1:1,000) antibodies (Cells Signaling Technology), acetylated α-tubulin (T7451, 1:4,000) and α-tubulin antibodies (T6074, 1:4,000) (Sigma Co., USA) and MEC17 (ABCAM: ab58742, 1:1,000). SP1 inhibitor Mithramycin, p38 inhibitor SB202190, JNK inhibitor SP600125 and HDAC6 specific inhibitor Tubastatin A (TBSA) were purchased from Selleckchem or synthesized in house. Nocodazole, Taxol and Lipopolysaccharide (LPS) were purchased from Sigma Co. Cell culture The macrophage cell line RAW264.7 (ATCC) was cultured in DMEM (GIBCO) supplemented with 10% FBS, pen/strep 100 U ml −1 and streptomycin 100 U ml −1 , and maintained in humidified incubators at 37 °C with 5% CO 2 . Macrophages were seeded into six-well plate (1 × 10 6 cells per well) and were stimulated by LPS (1 μg ml −1 ) the next day. Cell culture supernatant and cells lysates were collected at indicated time points and stored at −70 °C prior to analysis. Plasmids and shRNA Two HDAC6 shRNA sequences (no. 321323: 5′-GCTGACTACATTGCTGCTTT-3′ and no. 321357: 5′-CCTTGCTGGTGGCCGTATTAT-3′) were transduced by lentivirus into macrophages (Raw264.7 cell line) to establish stable HDAC6 KD macrophages. For MEC17 KD stable macrophages, two MEC17 shRNA sequences (no. 4781: 5′-GAGACATTAAGCCATACTCTT-3′ and no. 4864: 5′-GTGAACAACTTT GTCATCTTT-3′) were used through lentiviral transduction. pBabe-puro-HDAC6 plasmids and pCDNA-EGFP-tubulin plasmids were described previously [7] , [23] . Real-time RT–PCR Total RNA was extracted from the cells using Trizol reagent (Invitrogen, Carlsbad, CA) according to the manufacturer instructions. Two micrograms of total RNA from each sample were reverse transcribed to cDNA using Random primers and M-MLV Reverse Transcriptase. The cDNA product (2.0 μl) was used for quantitative PCR by using SsoFast EvaGreen Supermix kit (NO.172-5201, Bio-Rad). The primers were used as below: IL-10; 5′-GCTGAGGCGCTGTCATCGATTT-3′ and 5′-GGCCCTGCAGCTCTCAAGTGT-3′; GAPDH (internal control), 5′-ACAACTTTGGCATTGTGGAAG-3′ and 5′-GTTGAAGTCGCAGGAGACAAC-3′. Enzyme-linked immunosorbent assay The ELISA for detecting IL-10, TNF alpha, IL-6 and IL-1beta in cell culture supernatant and cell lysates was carried out in 96-well plate according to the manufacturer’s instruction (R&D Systems) using a plate reader at 450 nm. The concentration of each cytokine was determined according to the standard provided with the kits. Final values were normalized to total protein concentration. Western blotting analysis After treatment, cells were washed twice with cold PBS and then lysed in ice-cold NETN buffer (50 mM Tris-Cl (pH 7.4), 150 mM NaCl, 1 mM EDTA, 1% NP-40, 0.5% sodium deoxycholate, 1 mM sodium orthovanadate, 1 mM sodium fluoride, 1 mM phenylmethanesulfonylfluoride, 0.2 mM leupeptin, protease inhibitor cocktail (Sigma). Lysates were cleared by centrifugation (13,000 r.p.m. for 20 min). Protein concentrations were determined using the BCA assay (Pierce). Equal amounts of cell extracts were then resolved by SDS-PAGE, transferred to nitrocellulose membranes and probed with antibodies. Blots were detected using an ECL system (Amersham). Immunostaining Macrophages were treated with LPS for indicated times,fixed with 4% formaldehyde in PBS for 20 min and then permeabilized with 0.1% Triton-x-100 in PBS for 5 min at room temperature. Cells were blocked with 5% normal goat serum in PBS and incubated with anti-Ac-tubulin (1:1,000 dilution) overnight at 4 °C, followed by Alexa Fluor 488 goat anti-mouse IgG for 30 min. Nuclei was identified using DAPI staining. Immunostaining images were obtained using a Zeiss Axioskop compound microscope (Carl Zeiss). Animal experiments Male C57BL/6 mice (6–8 weeks) were used in all studies. All mice were housed at the Duke University mouse facilities and all procedures were approved by the Institutional Animal Care and Use Committee. HDAC6-specific inhibitor TBSA was dissolved in dimethyl sulfoxide (DMSO) and delivered by daily intraperitoneal (i.p.) injection at 0.5 mg per kg for 7 days. For serum cytokines assay, mice were injected with PBS or LPS (50 μg per mouse) by i.p. after 7 days of TBSA injection. Blood samples ≥0.5 ml were harvested at 4 h after LPS injection through the retro-orbital sinus with the tip of a Pasteur pipette. Blood samples in sealed tube were plated on ice during the experiment and then in cold room overnight to allow clot formation and retraction. Serum was harvested after centrifugation (5,000 g ) and stored at −80° for cytokine assay by ELISA. For LPS-induced lethality, mice were injected with PBS or LPS (5 mg per kg) by i.p. after 7 days TBSA (0.5 mg per kg) injection. In the first 10 h after LPS injection, mice survival was observed every 2 h with follow-up observations every 10 h. Statistical analysis Student’s t -tests were applied for comparisons. All data are expressed as mean±s.e.m. The significance threshold was at a level of 5% (* P <0.05; ** P <0.01). All the experiments were repeated three times. How to cite this article: Wang, B. et al. Microtubule acetylation amplifies p38 kinase signalling and anti-inflammatory IL-10 production. Nat. Commun. 5:3479 doi: 10.1038/ncomms4479 (2014).